Snail1-dependent control of embryonic stem cell pluripotency and lineage commitment Embryonic stem cells (ESCs) exhibit the dual properties of self-renewal and pluripotency as well as the ability to undergo differentiation that gives rise to all three germ layers. Wnt family members can both promote ESC maintenance and trigger differentiation while also controlling the expression of Snail1, a zinc-finger transcriptional repressor. Snail1 has been linked to events ranging from cell cycle regulation and cell survival to epithelial–mesenchymal transition (EMT) and gastrulation, but its role in self-renewal, pluripotency or lineage commitment in ESCs remains undefined. Here we demonstrate using isogenic pairs of conditional knockout mouse ESCs, that Snail1 exerts Wnt- and EMT independent control over the stem cell transcriptome without affecting self-renewal or pluripotency-associated functions. By contrast, during ESC differentiation, an endogenous Wnt-mediated burst in Snail1 expression regulates neuroectodermal fate while playing a required role in epiblast stem cell exit and the consequent lineage fate decisions that define mesoderm commitment. Embryonic stem cells (ESCs) exhibit the dual properties of self-renewal and pluripotency in tandem with an ability to express the zinc-finger transcriptional repressor, Snail1 (refs 1 , 2 , 3 ). Classically characterized as an inducer of the epithelial–mesenchymal transition (EMT) programs associated with early development, more recent studies suggest broader roles for Snail1 in regulating key functions in ESCs, mesenchymal stem cells, inducible pluripotent stem cells as well as cancer stem cells [4] , [5] , [6] , [7] , [8] , [9] . Efforts to link Snail1 functions solely to core stem cell properties such as self-renewal and phenotype plasticity have, however, proven problematic. First, while Snail1 expression can be regulated by the canonical Wnt pathway [10] , [11] , [12] , this signalling programme has been linked to apparently diametrically opposing roles in promoting ESC self-renewal versus triggering ESC differentiation [13] , [14] . Second, though Snail1 expression has been linked to events ranging from cell cycle regulation and cell survival to EMT [15] , [16] , its role in self-renewal, pluripotency or lineage commitment in mammalian ESCs remains undefined. Independent of the function of Snail1 in stem cell-associated developmental processes, ESCs have also been shown to share transcriptional signatures with cancer stem cells [17] , [18] , [19] , [20] . These studies have led to the suggestion that the properties of self-renewal and lineage commitment central to ESC function may be co-opted by discrete populations of cancer cells (that is, cancer stem cells or tumour initiating cells) to drive tumour growth, invasion and metastasis [9] , [21] , [22] , [23] , [24] , [25] , [26] . Though normal and neoplastic stem cells are both capable of expressing Snail1 (refs 1 , 2 , 3 , 4 , 5 , 6 , 7 , 8 , 9 , 23 , 25 ), the two cell types display disparate phenotypes. Ground-state ESCs are distinctly epithelial in character and express high levels of the cell adhesion molecule, E-cadherin [1] , [2] , [3] . Likewise, during somatic cell reprogramming to induced pluripotent stem cells, the multistep process necessarily involves a mesenchymal-to-epithelial transition [7] , [8] . By contrast, Snail1 as well as related EMT-inducing transcription factors (for example, Snail2, Twist1, Twist2, Zeb1 and Zeb2) reportedly confer cancer cells with mesenchymal cell-like characteristics more similar to those associated with EMT programs [9] , [15] , [16] , [21] , [22] , [23] , [24] , [25] , [26] . To date, attempts to reconcile these differences have been hampered by the paucity of available information regarding the role of endogenous Snail1 in normal stem cells. Given the ability of cultured ESCs to serve as a malleable platform for analysing Wnt-regulated self-renewal, pluripotency, EMT and germ layer commitment [1] , [2] , [3] , coupled with the proposed transcriptional overlap between ESCs and cancer stem cells [17] , [18] , [19] , [20] , we reasoned that Snail1 functions would be best assessed by targeting Snail1 in ground state as well as differentiating ESCs. To this end, we now describe the generation and characterization of isogenic pairs of Snail1 conditional knockout mouse ESCs. Herein, we demonstrate that Snail1 exerts Wnt-independent control over the ECS transcriptome without affecting stem cell self-renewal or pluripotency. Alternatively, during ESC differentiation, a Wnt-initiated burst in Snail1 expression is shown to play a required role in driving epiblast exit and the consequent lineage fate decisions that define neuroectodermal, endodermal and mesodermal commitment. Taken together, these data classify Snail1 as a transcriptional regulator that is expressed throughout the ESC life cycle—in both ground state as well as differentiating cells—where it exerts EMT-dependent as well as -independent control over cellular functions distinct from those assigned to cancer stem cells. Naive ESCs express Snail1 EMT-inducing transcription factors, including Snail1, have been proposed to confer expressing cells with ESC-like properties [9] , [21] , [22] , [23] , [24] , [25] , [26] . As such, we first sought to determine whether Snail1 is expressed in ESCs in vivo or in vitro , and if so, the functional ramifications of its generation. To this end, a Snai1 LacZ/+ mouse line was generated and blastocysts recovered from transgenic mice. LacZ staining, indicative of Snail1 expression, was detected in the inner cell mass (ICM) of E3.5 blastocyst stage embryos ( Fig. 1a left). Similarly, LacZ expression was confirmed in Snai1 LacZ/+ ESCs cultured in vitro under standard stem cell conditions ( Fig. 1a right). The heterogeneous expression of Snail1 expression in vitro is not related to the presence of primitive endoderm (PE)-like population as the PE markers, Sox17 and Gata6, were undetectable under these culture conditions ( Supplementary Fig. 1a ). 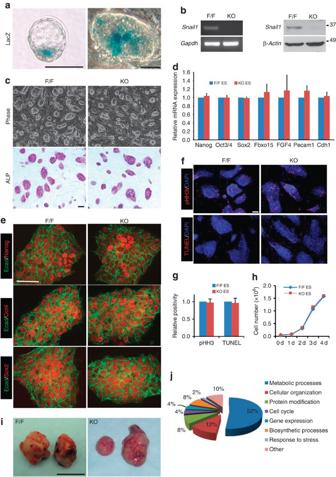Figure 1: Snail1 is expressed in ESCs but dispensable for pluripotency maintenance and growth. (a) LacZ staining ofSnai1LacZ/+E3.5 blastocyst ICM (left) and anin vitroculturedSnai1LacZ/+ESC colony (right). Bar, 0.1 mm. (b) RT–PCR (left) and western blot (right) of Snail1 expression in control (F/F) and knockout (KO) ESCs. Results are representative of three or more experiments performed. (c) Phase contrast (top) and alkaline phosphatase staining (AP, bottom) of F/F and KO ESCs. All F/F colonies are AP-positive. All colonies (that is, 100±0%) were AP-positive (mean±1 s.d.;n=5) and the ratio of AP staining intensity in control to KO cells was 1.00:0.98±0.09 (mean±1 s.d.;n=3). Bar, 100 μm. (d) mRNA expression of pluripotent genes (Nanog,Oct3/4andSox2) and ESC-specific genes (Fbxo15,Fgf4andPecam1) as well as E-cadherin (Cdh1) in control and KO ESCs as assessed by real-time PCR (mean±1s.d.;n=3). (e) Immunofluorescence of pluripotent markers (Nanog,Oct4, andSox2) and E-cadherin in F/F and KO ESCs as assessed by confocal microscopy. Results are representative of three or more experiments. Quantification of immunofluorescence staining of each panel is shown inSupplementary Table 3and is representative of five or more experiments performed. Bar, 100 μm. (f) Phospho-histone H3 (pHH3) (top) and TUNEL staining (bottom) of F/F and KO ESCs. Bar, 100 μm. (g) Quantification of pHH3 and TUNEL staining of F/F and KO ESCs (mean±1 s.d.;n=3). (h) Growth rate assay of F/F and KO ESCs cultured atop feeder layers (mean±1 s.d.;n=3). (i) Teratomas formed by F/F and KO ESCs 6 weeks after injection. No significant differences in teratoma size or weight were observed (six mice in each group). Bar, 1 cm. (j) GO categories altered between F/F and KO ESCs using a minimum cutoff of twofold change. The full GO category analysis with statistical evaluation is presented inSupplementary Data 1. Figure 1: Snail1 is expressed in ESCs but dispensable for pluripotency maintenance and growth. ( a ) LacZ staining of Snai1 LacZ/+ E3.5 blastocyst ICM (left) and an in vitro cultured Snai1 LacZ/+ ESC colony (right). Bar, 0.1 mm. ( b ) RT–PCR (left) and western blot (right) of Snail1 expression in control (F/F) and knockout (KO) ESCs. Results are representative of three or more experiments performed. ( c ) Phase contrast (top) and alkaline phosphatase staining (AP, bottom) of F/F and KO ESCs. All F/F colonies are AP-positive. All colonies (that is, 100±0%) were AP-positive (mean±1 s.d. ; n =5) and the ratio of AP staining intensity in control to KO cells was 1.00:0.98±0.09 (mean±1 s.d. ; n =3). Bar, 100 μm. ( d ) mRNA expression of pluripotent genes ( Nanog , Oct3/4 and Sox2 ) and ESC-specific genes ( Fbxo15 , Fgf4 and Pecam1 ) as well as E-cadherin (Cdh1) in control and KO ESCs as assessed by real-time PCR (mean±1s.d. ; n =3). ( e ) Immunofluorescence of pluripotent markers ( Nanog , Oct4 , and Sox2 ) and E-cadherin in F/F and KO ESCs as assessed by confocal microscopy. Results are representative of three or more experiments. Quantification of immunofluorescence staining of each panel is shown in Supplementary Table 3 and is representative of five or more experiments performed. 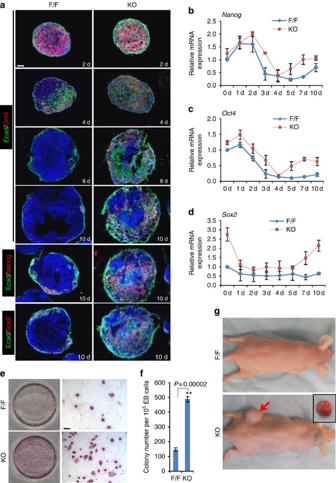Figure 3: Snail1-deleted ESCs retain pluripotent potential during differentiation. (a) F/F and KO EBs were cultured for 2–10 d and E-cadherin expression monitored in tandem with Oct4, Nanog or Sox2 by immunofluorescence. Results are representative of three or more experiments. Bar, 200 μm. (b–d) Real-time PCR ofNanog,Oct4andSox2expression in F/F or KO EBs as a function of time (mean±1 s.d.,n=3). ANOVA analyses are presented inSupplementary Table 3. (e,f) F/F and KO cells were dissociated from 10-d-old EBs and re-cultured atop feeder layers in stem cell culture media to induce colony re-formation and then stained for ALP activity (pink). The numbers of ALP-positive colonies are quantified as the mean±1 s.d. (n=3) **P<0.01; Student’st-test. Bar, 100 μm. (g) 106F/F or KO cells were dissociated from 10-d-old EBs and subcutaneously injected into nude mice (three mice in each group). Only KO cells formed teratomas (indicated by arrow) after a 2-month growth period. Bar, 100 μm. ( f ) Phospho-histone H3 (pHH3) (top) and TUNEL staining (bottom) of F/F and KO ESCs. Bar, 100 μm. ( g ) Quantification of pHH3 and TUNEL staining of F/F and KO ESCs (mean±1 s.d. ; n =3). ( h ) Growth rate assay of F/F and KO ESCs cultured atop feeder layers (mean±1 s.d. ; n =3). ( i ) Teratomas formed by F/F and KO ESCs 6 weeks after injection. No significant differences in teratoma size or weight were observed (six mice in each group). Bar, 1 cm. ( j ) GO categories altered between F/F and KO ESCs using a minimum cutoff of twofold change. The full GO category analysis with statistical evaluation is presented in Supplementary Data 1 . Full size image To next assess the functional consequences of Snail1 expression in ESCs, a 4-hydroxytamoxifen (4-OHT)-inducible Snai1 fl/fl ; CAG-Cre+ conditional knockout allele was generated. Following incubation of Snai1 fl/fl ; CAG-Cre+ ESCs with 4-OHT for 2 days, Snai1 deletion was confirmed at both the mRNA and protein levels ( Fig. 1b ). To determine the impact of Snail1 deletion on ESC self-renewal, untreated Snai1 fl/fl ; CAG-Cre+ ESCs (herein referred to as ‘F/F’ or ‘control’) and the 4-OHT-treated Snai1 fl/fl ; CAG-Cre+ ESCs (referred to as ‘KO’) were cultured for >20 passages under standard ESC conditions atop fibroblast feeder layers in the presence of exogenous LIF. Following Snail1 deletion, neither ESC morphology, alkaline phosphatase staining, E-cadherin distribution nor pluripotent marker expression were affected as assessed by real-time PCR or immunofluorescence ( Fig. 1c–e ; PCR primer sequences are included in Supplementary Table 1 ). While Snail1 expression has also been linked to cell cycle and cell survival regulation [16] , no differences in ESC proliferation, phospho-histone H3 or TUNEL staining were observed between control and KO ESCs ( Fig. 1f–h ). Finally, consistent with the conclusion that Snail1-deleted ESCs retain pluripotent potential, both control F/F and KO ESCs supported teratoma formation to an equivalent degree in vivo ( Fig. 1i ). Given the inability of Snail1 deletion to affect ESC morphology, E-cadherin expression, self-renewal, proliferation, apoptosis or pluripotent potential, we considered the possibility that Snail1 might be inoperative in ESCs as a consequence of the potential absence of required co-transcriptional modifiers or post-transcriptional modification [15] , [16] . Indeed, though Wnt proteins can maintain ESCs in a naive state [13] , [14] , [27] , [28] , [29] , [30] , [31] , [32] , [33] , [34] and Snail1 expression is regulated by a canonical Wnt-GSK3 pathway [3] , [10] , [11] , [12] , neither the addition of exogenous Wnt3a nor inhibition of endogenous Wnt secretion with the Porcupine inhibitor, IWP2 (ref. 35 ), significantly affected Snail1 protein levels ( Supplementary Fig. 1b ). These results do not necessarily reflect the operation of non-canonical Wnt signalling cascades [13] , [14] , [27] , [28] , [29] , [30] , [31] , [32] , [33] , [34] or defects in Snail1 expression as exogenous Wnt3a induced the canonical target, Axin2 , while Snail1 levels increased following GSK3 inhibition [10] , [12] , [15] , [16] ( Supplementary Fig. 1c ). Likewise, when ESC culture conditions were switched from LIF-supplemented, serum-containing media to a serum-free, 2i media (that is, CHIR and MEK inhibitors) to enrich for naive ESCs [36] , the expression of the specific stem cell markers, Fgf4 , Fbxo15 and Rex1 , were upregulated comparably in control and Snail KO cultures despite the enhanced expression of Snai1 in the control ESCs ( Supplementary Fig. 1d,e ). As Snail1 expression was insensitive to endogenous or exogenous Wnt and failed to repress E-cadherin in naive ESCs, we next considered the possibility that the transcription factor was held in inactive state [15] , [16] . Hence, control and KO ESCs were harvested from LIF-supplemented, fibroblast feeder layers and gene expression was profiled. 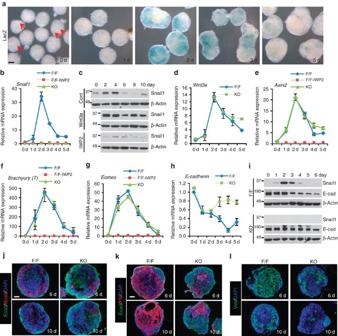Contrary to expectations, >350 transcripts were differentially expressed between the control and KO isogenic ESC pairs ( Supplementary Data 1 ). Figure 2: Snail1 expression is mediated by Wnt signalling and critical for EMT during ESC cell differentiation. (a) LacZ staining highlighting the dynamic expression of Snail1 during EB differentiation ofSnai1LacZ/+ESCs. Only small subsets of cells express Snail1 in EBs at day 0 (red arrows). Results are representative of three or more experiments performed at each time point. Bar, 300 μm. (b,c) Real-time PCR and western blot analyses of Snail1 expression patterns by either F/F or KO EBs in the absence or presence of IWP2 or Wnt3a. Results are representative of three or more experiments (error bars depict mean±1 s.d.). Quantification of western blot data is included inSupplementary Table 2. (d–g) IWP2, but not Snail1 deletion, blocks primitive streak gene expression as assessed byAxin2,Brachyury,EmoesmRNA levels. Results are presented as the mean±1 s.d. of 3 experiments (error bars depict mean±1 s.d.). (h,i) Relative E-cadherin expression during F/F and KO EB differentiation. Real-time PCR data are shown as the mean±1 s.d. of three experiments and western blot quantification (results are representative of three experiments) are shown inSupplementary Table 3. (j–l) Dual immunofluorescence of E-cadherin in tandem with either N-cadherin, fibronectin or vimentin at 6 d and 10 d of EB culture. Bar, 200 μm. Gene ontology identified multiple changes in regulatory networks, but none of the top 20 most significantly regulated GO processes impacted pathways central to stem cell self-renewal, pluripotency or EMT ( Supplementary Table 2a ). Interestingly, 14 of the 20 top GO processes affected by Snail1 deletion were largely confined to the regulation of programs central to cellular protein metabolism, cellular nitrogen compound metabolism and nucleic acid-related metabolic processes ( Fig. 1j and Supplementary Table 2a ). Hence, while Snail1 impacts ESC transcriptional programs, it does not play a required role in self-renewal or pluripotent potential. Snail1-dependent control of EB differentiation In the absence of LIF, ESCs cultured as suspended aggregates or EBs undergo Wnt-dependent self-organization and axis formation while generating descendants of all three germ layers [2] , [3] . Under these conditions, anteroposterior polarity is established and a primitive streak-like region is formed where cells undergo EMT and generate mesodermal progenitors [3] , [37] . Using EBs generated from Snai1 LacZ/+ ESCs, the reporter displayed a dynamic expression profile with peak activity observed between days 2 and 3 ( Fig. 2a ). Likewise, Snail1 mRNA and protein expression levels increased slowly from day 0, peaked at day 2, and then diminished abruptly ( Fig. 2b,c ). Unlike ESCs, Snail1 expression in EBs was dependent entirely on Wnt signalling as Snail1 mRNA and protein levels fell to background levels in the presence of IWP2 while Snail1 levels were stabilized at peak levels in the presence of exogenous Wnt3a ( Fig. 2b,c ). Figure 2: Snail1 expression is mediated by Wnt signalling and critical for EMT during ESC cell differentiation. ( a ) LacZ staining highlighting the dynamic expression of Snail1 during EB differentiation of Snai1 LacZ/+ ESCs. Only small subsets of cells express Snail1 in EBs at day 0 (red arrows). Results are representative of three or more experiments performed at each time point. Bar, 300 μm. ( b , c ) Real-time PCR and western blot analyses of Snail1 expression patterns by either F/F or KO EBs in the absence or presence of IWP2 or Wnt3a. Results are representative of three or more experiments (error bars depict mean±1 s.d.). Quantification of western blot data is included in Supplementary Table 2 . ( d – g ) IWP2, but not Snail1 deletion, blocks primitive streak gene expression as assessed by Axin2 , Brachyury , Emoes mRNA levels. Results are presented as the mean±1 s.d. of 3 experiments (error bars depict mean±1 s.d.). ( h , i ) Relative E-cadherin expression during F/F and KO EB differentiation. Real-time PCR data are shown as the mean±1 s.d. of three experiments and western blot quantification (results are representative of three experiments) are shown in Supplementary Table 3 . ( j – l ) Dual immunofluorescence of E-cadherin in tandem with either N-cadherin, fibronectin or vimentin at 6 d and 10 d of EB culture. Bar, 200 μm. Full size image Coincident with the increase in Snail1 expression during EB differentiation, endogenous Wnt3a and the canonical Wnt target, Axin2 (refs 3 , 12 ), were induced along with the primitive streak markers, brachyury ( T ) and Eomes ( Fig. 2d–g ) [38] , [39] . Concurrently, EMT was initiated as reflected by decreasing levels of E-cadherin mRNA followed by similar losses at the protein level ( Fig. 2h,i ). As expected [2] , [3] , in the presence of IWP2, expression of the primitive streak markers, Axin2 , T and Eomes , was suppressed completely ( Fig. 2e–g ). To determine the degree to which Snail1 participates in Wnt-dependent EB differentiation, Snail1 KO EBs were generated and cultured over a 5–10-d time course. In contrast to Wnt-inhibited EBs, the Snail1-deleted EBs activated Wnt3a and Axin2 expression comparably to control EBs ( Fig. 2d,e ). Further, expression of T and Eomes were unaffected in the absence of Snail1 ( Fig. 2f,g ). Hence, although Wnt is the dominant inducer of Snail1 expression ( Fig. 2b,c ), Wnt-dependent primitive streak initiation proceeds independently of Snail1 expression, a finding consistent with normal T expression in Snail1 KO mice [40] . Nevertheless, Snail1 proved essential for driving a full EMT programme as the normal losses in E-cadherin mRNA and protein expression levels observed during control EB differentiation were blunted significantly in Snail1 KO EBs ( Fig. 2h,i ). As assessed alternatively by immunofluorescence, while residual E-cadherin expression was largely confined to the PE layer in control EBs after 6–10 days in culture, residual E-cadherin was distributed throughout the interior of the KO EBs ( Fig. 2j–l ). In concert with the blunted downregulation of E-cadherin observed in Snail1 KO EBs, the distribution of the mesenchymal cell markers, N-cadherin, fibronectin and vimentin, whose expression are normally upregulated during differentiation [2] , [3] , were also decreased markedly relative to control F/F EBs ( Fig. 2j–l ). Snail1 deletion did not, however, completely ablate decreases in E-cadherin expression, or sustain an absolute block in the induction of the mesenchymal markers ( Fig. 2j–l ), suggesting the existence of potential compensatory changes in other EMT-inducing factors. Indeed, while ablating Wnt signalling with IWP2 effectively inhibited Snai1 , Slug/Snai2 , Twist1 and Twist2 (but not Zeb1 or Zeb2 expression), Snail1 KO EBs only displayed partial losses in Slug , Twist2 , Zeb1 and Zeb2 expression ( Supplementary Fig. 2a ). As recent studies indicate that the ability of Wnt inhibitors to perturb EB differentiation can be bypassed by blocking GSK3 activity [41] , we compared the ability of the GSK3 inhibitor, CHIR99021, to rescue the expression of EMT-associated transcription factors in IWP2-treated control versus Snail1 KO EBs. Interestingly, the loss of Snai1 , Slug/Snai2 , Twist1 or Twist2 expression in IWP2-treated control EBs, as well as the blunted ability of Snail1 KO EBs to express Slug/Snail2 , Twist1 or Twist2 , could be rescued by inhibiting GSK3 activity alone ( Supplementary Fig. 2b ). Though Snail1 has been proposed to act as an upstream regulator of the asynchronous patterns of Slug, Twist1 and Zeb1 expression [1] , [42] , [43] , [44] , [45] , these findings suggest that the Wnt-dependent control of GSK3 activity, rather than Snail1 expression per se , plays a dominant role in regulating Slug/Snail2 , Twist1 , Twist2 and Zeb1 expression in differentiating EBs. In tandem with EMT-associated defects in Snail1 KO EBs, recent studies suggest that Snail1 also functions as a critical cell survival and motility factor [15] , [16] . However, both control and KO EBs proliferated at equivalent rates, and significant differences in apoptosis were not detected ( Supplementary Fig. 3a,b ). To alternatively evaluate potential roles for Snail1 in controlling motility during ESC differentiation, 3-d-old EBs were isolated (a time point at which Snail1 protein expression has peaked), and cultured atop gelatin-coated dishes in differentiation media. Under these conditions, no significant differences in cell migration were observed in control versus KO EBs over the next 48 h period, a finding consistent with ability of Snail1-deleted fibroblasts to maintain full motile activity [46] ( Supplementary Fig. 3c ). During this time frame, E-cadherin staining levels were also comparable between control and KO cells migrating from the EB edge ( Supplementary Fig. 3d ). Motility changes between control and KO EBs were, however, detected after a 72-h culture period, but only after E-cadherin levels were more extensively reduced in the Snail1 + EBs ( Supplementary Fig. 3d ). The inability of Snail1 to affect cell migration was also confirmed in wound-healing assays ( Supplementary Fig. 3e,f ). Hence, Snail1 does not appear to play a major role in regulating cell growth, apoptosis or the early motility responses associated with EB differentiation. Pluripotent potential is retained in Snail1 KO EBs As ESCs are both E-cadherin- and Oct4-positive [1] , [2] , [3] , the inability of Snail1 KO EBs to respond to Wnt signalling by downregulating E-cadherin is equally consistent with a specific defect in EMT or a broader defect in controlling ESC exit from the pluripotent state. In 2-d-old control EBs, all cells maintain an E-cad + /Oct4 + phenotype, but gradually decrease E-cadherin and Oct4 expression as a function of time, save for the outer rim of extra embryonic primitive/visceral endoderm-like cells [47] ( Fig. 3a ). By contrast, in Snail1 KO EBs, large numbers of E-cadherin + /Oct4 + are maintained throughout these structures, even after a 10-d differentiation period ( Fig. 3a ). Consistent with these findings, Nanog and Sox2 were likewise expressed at increased levels in the 10-d-old Snail1 KO EBs ( Fig. 3a ). Though quantitative analyses of Oct4 , Nanog and Sox2 mRNA levels during differentiation of control and KO EBs are complicated by the heterogeneous pattern of pluripotent marker expression in the Snail1-deleted population, qPCR analyses confirmed consistently higher levels of each transcription factor in the KO population ( Fig. 3b–d ). To assess whether the continued expression of Oct4 , Nanog and Sox2 in KO EBs reflects functional pluripotency, cells were dissociated from 10-d-old control or Snail1 KO EBs, and re-cultured atop feeder cells under standard ESC culture conditions. As predicted, the number of pluripotent colonies (as assessed by alkaline phosphatase staining) was increased almost fivefold in the cell populations recovered from KO EBs ( Fig. 3e ). Additionally, when cells recovered from 10-d-old control EBs were injected into nude mouse recipients, no teratomas were generated (0/3). By contrast, 2/3 injected sites formed teratomas when animals were inoculated with cells isolated from KO EBs ( Fig. 3g ). Similarly, when a more sensitive assay system was employed using control and KO EBs embedded in Matrigel [48] and injected into NOD scid gamma mice, teratoma mass was increased fourfold in the KO tissues ( Supplementary Fig. 4 ). Hence, in contrast to current models proposed for cancer cells wherein Snail1 and associated EMT factors lend expressing cells stem-like characteristics [9] , [21] , [22] , [23] , [24] , [25] , [26] , endogenous Snail1 drives EMT programs in pluripotent stem cells that trigger the loss of pluripotency and self-renewal potential. Figure 3: Snail1-deleted ESCs retain pluripotent potential during differentiation. ( a ) F/F and KO EBs were cultured for 2–10 d and E-cadherin expression monitored in tandem with Oct4, Nanog or Sox2 by immunofluorescence. Results are representative of three or more experiments. Bar, 200 μm. ( b – d ) Real-time PCR of Nanog , Oct4 and Sox2 expression in F/F or KO EBs as a function of time (mean±1 s.d., n =3). ANOVA analyses are presented in Supplementary Table 3 . ( e , f ) F/F and KO cells were dissociated from 10-d-old EBs and re-cultured atop feeder layers in stem cell culture media to induce colony re-formation and then stained for ALP activity (pink). The numbers of ALP-positive colonies are quantified as the mean±1 s.d. ( n =3) ** P <0.01; Student’s t -test. Bar, 100 μm. ( g ) 10 6 F/F or KO cells were dissociated from 10-d-old EBs and subcutaneously injected into nude mice (three mice in each group). Only KO cells formed teratomas (indicated by arrow) after a 2-month growth period. Full size image Snail1 drives Wnt-dependent EpiSC exit The retention of pluripotent cells in Snail1 KO EBs can be potentially ascribed to the presence of ESCs, epiblast stem cells (EpiSCs), or embryonic germ cells [49] , [50] , [51] . To further define the pluripotent cell population that accumulated in Snail1 KO EBs, gene expression profiles were obtained for 5-d-old control and KO EBs ( Supplementary Data 2 ). Interestingly, while gene signatures associated with ESCs or embryonic germ cells were not altered between control and Snail1 KO EBs, EpiSC-specific genes were upregulated dramatically in Snail1 KO EBs ( Fig. 4a ). In confirmation of the gene microarray results, real-time PCR demonstrated that expression of multiple epiblast-associated transcripts (for example, Fgf5 , Claudin6 , Otx2 and Dnmt3b [13] ) were upregulated significantly in Snail1 KO EBs ( Fig. 4b ). By contrast, expression levels of stem cell-associated genes that are primarily expressed in ESCs, but not epiblasts (for example, Fbxo15 , FGF4 , Pecam1 and Rex1 ) [52] , were downregulated comparably in both control and KO EBs relative to ESCs ( Fig. 4c ). These data support a model wherein Snail1 deficiency does not affect the transition of ESCs to EpiSCs (a process usually limited to the first 2 days of EB culture [3] ), but rather maintains epiblast-associated transcripts at high levels ( Fig. 4d ). Defects in the ability of Snail1 KO EBs to effectively transit through the epiblast stage phenocopies Wnt3-null embryos as well as EBs wherein Wnt signalling has been silenced, yielding stem cell populations that fail to differentiate beyond the epiblast stage [13] , [53] . Indeed, IWP2-treated EBs that are incapable of expressing Snai1 likewise maintained FGF5 expression at elevated levels ( Fig. 4d ). In further support of the conclusion that the pluripotent stem cells retained in KO EBs are epiblast/epiblast-like in origin, cells were co-stained for Pecam1 and Oct4. Whereas ESCs are Pecam1 + /Oct4 + , Pecam1 expression shifts to mesoderm-derived endothelial cells in maturing EBs while EpiSCs express Oct4 + alone [49] , [50] . As predicted, KO EBs display markedly increased numbers of Oct4 + /Pecam1 − epiblast-like stem cells ( Fig. 4e ). Further, when WT and KO ESCs were cultured directly under EpiSC-inducing conditions [13] , both populations displayed a similar ability to undergo EpiSC differentiation as assessed by morphology, AP activity and gene expression ( Fig. 4f,g ). Hence, Snail1 does not play a required role in generating EpiSCs, but rather serves as a critical transducer of the Wnt-initiated signals required for epiblast differentiation. Using Snail1 over-expressing ESC lines, recent studies have suggested that Snail1 may control ESC differentiation by targeting miR200 family members [5] , [6] . However, while 3-d-old Snail1 KO EBs display marked changes in miRNA expression patterns, significant alterations in the miR200 family were not yet detected at this time point ( Supplementary Fig. 5a–c ) [54] . 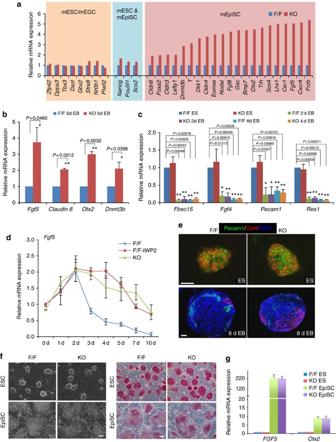Figure 4: Snail1 regulates epiblast exit during ESC differentiation. (a) Normalized gene expression values (as determined from a single representative gene microarray) were obtained from 5-d-old control versus KO EBs. F/F and KO EBs display similar expressions level for mouse ESC and embryonic germ cell-associated genes while KO EBs express higher levels of EpiSC-associated genes. (b) Real-time PCR of the EpiSC markers (Fgf5,Claudin6,Otx2andDnmt3b) in F/F versus KO EBs (mean±1 s.d.;n=3). *P<0.05, **P<0.01; Student’st-test. (c) Comparison of expression levels by real-time PCR of ESC-specific genes (Fbxo15,FGF4,Pecam1andRex1) in F/F versus KO ESCs and EBs at 2 and 4 d of culture (mean±1 s.d.;n=3). *P<0.05, **P<0.01; Student’st-test. (d) Fgf5expression during EB differentiation as assessed by real-time PCR in F/F, IWP2-treated F/F or KO EBs. Results are shown as the mean±1 s.d. (n=3). (e) Pecam1 and Oct4 immunofluorescence in ESCs and 8-d-old EBs highlighting Pecam1 and Oct4 colocalization in ESCs, but not in EBs. Bar, 200 μm. (f) Phase contrast (left panels) and AP staining (right panels) demonstrate the comparable changes observed as ESCs transition to EpiSCs in the presence of FGF2 and Activin A between F/F and KO cells. Bar, 100 μm. (g) Real-time PCR of EpiSC markers (Fgf5andOtx2) during conversion of ESCs to EpiSCs in F/F versus KO cells (mean±1 s.d.;n=3). Figure 4: Snail1 regulates epiblast exit during ESC differentiation. ( a ) Normalized gene expression values (as determined from a single representative gene microarray) were obtained from 5-d-old control versus KO EBs. F/F and KO EBs display similar expressions level for mouse ESC and embryonic germ cell-associated genes while KO EBs express higher levels of EpiSC-associated genes. ( b ) Real-time PCR of the EpiSC markers ( Fgf5 , Claudin6 , Otx2 and Dnmt3b ) in F/F versus KO EBs (mean±1 s.d. ; n =3). * P <0.05, ** P <0.01; Student’s t -test. ( c ) Comparison of expression levels by real-time PCR of ESC-specific genes ( Fbxo15 , FGF4 , Pecam1 and Rex1 ) in F/F versus KO ESCs and EBs at 2 and 4 d of culture (mean±1 s.d. ; n =3). * P <0.05, ** P <0.01; Student’s t -test. ( d ) F gf5 expression during EB differentiation as assessed by real-time PCR in F/F, IWP2-treated F/F or KO EBs. Results are shown as the mean±1 s.d. ( n =3). ( e ) Pecam1 and Oct4 immunofluorescence in ESCs and 8-d-old EBs highlighting Pecam1 and Oct4 colocalization in ESCs, but not in EBs. Bar, 200 μm. ( f ) Phase contrast (left panels) and AP staining (right panels) demonstrate the comparable changes observed as ESCs transition to EpiSCs in the presence of FGF2 and Activin A between F/F and KO cells. Bar, 100 μm. ( g ) Real-time PCR of EpiSC markers ( Fgf5 and Otx2 ) during conversion of ESCs to EpiSCs in F/F versus KO cells (mean±1 s.d. ; n =3). Full size image Snail1-dependent control of germ layer commitment A partial loss in E-cadherin expression in Snail1 KO EBs suggests that portions of the EMT programme remain operative. Canonical Wnt signalling induces Flk1 expression throughout the posterior mesoderm where expressing cells give rise to hematopoietic, endothelial and cardiovascular progenitors [2] , [55] , but the role of endogenous Snail1 in these processes is unknown. As expected, blocking Wnt secretion with IWP2 inhibits all mesodermal differentiation programs as assessed by Flk1 , Pecam1 or Nkx2.5 expression ( Fig. 5a ) [2] , [3] . In agreement with the proposition that Snail1 serves as a critical downstream effector of Wnt-induced mesoderm commitment, Snail1 KO EBs display partial but significant defects in morphology as well as Flk1 , Pecam1 and Nkx2.5 expression ( Fig. 5a and Supplementary Fig. 6a ). Likewise, whereas Wnt inhibition predisposes EBs to commit to a neuroectodermal default pathway [2] , [3] , Snail1 KO EBs display a shift in neuroectodermal commitment in combination with marked defects in mesoderm- and endoderm-associated gene expression ( Fig. 5b , Supplementary Fig. 6b and Supplementary Table 2b ). Immunostaining for neuron-associated Tuj1 confirmed increased neuroectoderm formation in Snail1 KO EBs while mesoderm-associated Pecam1 and cTnT were decreased markedly ( Fig. 5c and Supplementary Fig. 6d ). In tandem with defects in mesoderm commitment, Snail1 KO EBs displayed an impaired ability to generate either vascular networks or beating EBs ( Fig. 5c and Supplementary Fig. 6c,e ). These defects in lineage commitment are not confined to the in vitro setting as gene expression profiling of control versus Snail1 KO teratomas revealed similar increases in neuroectodermal commitment with multiple defects in EMT pathways and mesoderm differentiation ( Supplementary Fig. 6f and Supplementary Data 3 ). 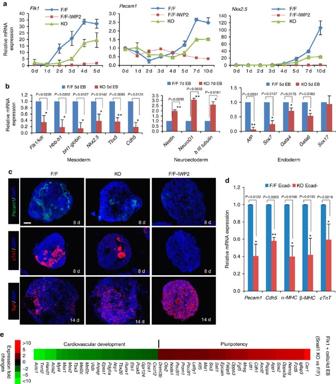Figure 5: Snail1-dependent regulation of germ layer commitment and differentiation. (a) Snail1 deletion reduces, while IWP2-dependent inhibition of Wnt signalling blocks, the expression of hematopoietic progenitor (Flk1), endothelial cell (Pecam1) and cardiomyocyte progenitor (Nkx2.5) differentiation markers (mean±1 s.d.;n=3). (b) Snail1 deletion inhibits mesodermal/endodermal while promoting neuroectodermal gene expression (mean±1 s.d.;n=3). *P<0.05, **P<0.01; Student’st-test. (c) Pecam1, cTnT and Tuj1 expression in F/F, IWP2-treated F/F and Snail1 KO EBs as assessed by immunofluorescence as a function of time. Results are representative of three or more experiments performed. Bar, 200 μm. (d) Real-time PCR of cardiovascular gene expression in E-cadherin-cells sorted from 8-d-old F/F and KO EBs (mean±1 s.d.;n=3). *P<0.05, **P<0.01; Student’st-test. (e) Heat map illustrating defects in cardiovascular gene expression with upregulated pluripotent gene expression in Flk1+cells sorted from 4-d-old Snail1 KO EBs relative to F/F EBs. Figure 5: Snail1-dependent regulation of germ layer commitment and differentiation. ( a ) Snail1 deletion reduces, while IWP2-dependent inhibition of Wnt signalling blocks, the expression of hematopoietic progenitor ( Flk1 ), endothelial cell ( Pecam1 ) and cardiomyocyte progenitor ( Nkx2.5 ) differentiation markers (mean±1 s.d. ; n =3). ( b ) Snail1 deletion inhibits mesodermal/endodermal while promoting neuroectodermal gene expression (mean±1 s.d. ; n =3). * P <0.05, ** P <0.01; Student’s t -test. ( c ) Pecam1, cTnT and Tuj1 expression in F/F, IWP2-treated F/F and Snail1 KO EBs as assessed by immunofluorescence as a function of time. Results are representative of three or more experiments performed. Bar, 200 μm. ( d ) Real-time PCR of cardiovascular gene expression in E-cadherin - cells sorted from 8-d-old F/F and KO EBs (mean±1 s.d. ; n =3). * P <0.05, ** P <0.01; Student’s t -test. ( e ) Heat map illustrating defects in cardiovascular gene expression with upregulated pluripotent gene expression in Flk1 + cells sorted from 4-d-old Snail1 KO EBs relative to F/F EBs. Full size image Given the shift to ectodermal as opposed to mesodermal differentiation, we next considered the possibility that defects in mesodermal marker gene expression arose indirectly as a consequence of decreasing the pool size of mesodermal progenitors (that is, due to the combined increase in epiblast-like and neuroectodermal-committed cell populations). To determine whether Snail1 directly controls mesoderm commitment and/or differentiation, cells that had successfully initiated EMT (that is, E-cadherin − cell populations) were recovered from 8-d-old control and KO EBs by cell sorting and monitored for defects in endothelial, hematopoietic or cardiovascular marker expression. Under these conditions, E-cadherin – cells isolated from KO EBs continued to display marked defects in mesoderm commitment, indicating that cells that successfully engaged an EMT programme nevertheless required Snail1 to complete normal differentiation ( Fig. 5d ). Likewise, when early mesoderm-committed Flk1 + cells were recovered from 4-d-old control versus KO EBs, gene expression profiling revealed a marked downregulation of transcripts associated with cardiovascular development in Snail1 KO Flk1 + cells in combination with the exaggerated expression of pluripotent markers ( Fig. 5e and Supplementary Data 4 ). Confirming a required role for Snail1 in Wnt-induced mesoderm commitment [2] , [3] , whereas GSK3 inhibition rescues the ability of IWP2-treated control EBs to upregulate Axin2 , Brachyury , Eomes , Pecam1 and Nkx2.5 expression, Snail1 KO EBs treated with IWP2 and CHIR99021 continued to display defects in Pecam1 and Nkx2.5 expression ( Supplementary Fig. 7a,b ). Late-stage Snail1 controls cardiomyocyte development Taken together, our data indicate that EMT-associated Snail1 expression plays a required role in determining neuroectodermal pool size as well as early mesodermal commitment and differentiation. However, even after the initial burst in Wnt signalling and Snail1 expression has diminished (that is, by day 4; see Fig. 2b ), EBs continue to dynamically re-activate canonical Wnt signalling (as assessed by Axin2 reporter activity) and Snail1 expression through days 7–15 ( Fig. 6a ). Given that the canonical Wnt cascade may continue to affect cell function following early lineage commitment decisions, 4-d-old post-EMT control EBs were either treated with IWP2 to block further Wnt signalling or treated with 4-OHT to delete Snail1 expression, and the culture period continued until d 8 ( Fig. 6b ). By delaying Wnt inhibition or Snail1 deletion, almost all cells downregulated early EB markers (monitored as E-cad + /Oct4 + cells) to a degree comparable to control EBs ( Fig. 6c ). However, as studies have demonstrated that late-stage inhibition of Wnt signalling promotes, rather than inhibits, cardiomyocyte development [56] , we considered the possibility that Wnt may repress cardiomyogenesis via a Snail1-dependent process. Indeed, the ability of late-stage Wnt inhibition to promote cardiomyocyte-associated gene expression was recapitulated by Snail1 deletion ( Fig. 6d,e ). Hence, mesoderm cell functions that are Wnt-regulated after lineage commitment decisions have been executed rely on Snail1 as a key downstream effector. 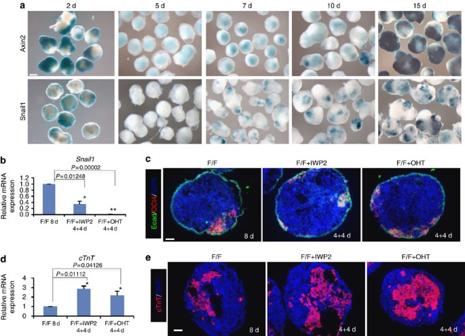Figure 6: Snail1-dependent control of mesoderm commitment. (a) LacZ staining of the canonical Wnt signalling reporter, Axin2, and Snail1 are downregulated after primitive streak formation at day 5, but reactivated at later stages of EB differentiation. Bar, 600 μm. (b) 4-d-old control F/F EBs were treated with IWP2 to block Wnt signalling or 4-OHT to delete Snail1, respectively, and EBs collected for assay at day 8. Real-time PCR confirms that Snai1 expression is significantly repressed by IWP2 or 4-OHT treatment. mRNA expression levels are reported as the mean ±1 s.d. (n=3).*P<0.05, **P<0.01; Student’st-test. Bar, 200 μm. (c) At the 4 d time point, neither IWP2 nor Snail1 excision interferes with stem cell exit from the pluripotent state as assessed by E-cadherin/Oct4 staining relative to untreated F/F controls. Bar, 200 μm. (d) Cardiomyocyte marker (cTnT) expression is upregulated at the RNA level following inhibition of Wnt signalling with IWP2 or Snail1 excision. cTnT mRNA expression levels are reported as the mean±1 s.d. (n=3). *P<0.05, **P<0.01; Student’st-test. Bar, 200 μm. (e) cTnT protein levels are upregulated following IWP2 treatment or Snail1 excision. Immunofluorescent images are representative of three experiments performed. Figure 6: Snail1-dependent control of mesoderm commitment. ( a ) LacZ staining of the canonical Wnt signalling reporter, Axin2, and Snail1 are downregulated after primitive streak formation at day 5, but reactivated at later stages of EB differentiation. Bar, 600 μm. ( b ) 4-d-old control F/F EBs were treated with IWP2 to block Wnt signalling or 4-OHT to delete Snail1, respectively, and EBs collected for assay at day 8. Real-time PCR confirms that Snai1 expression is significantly repressed by IWP2 or 4-OHT treatment. mRNA expression levels are reported as the mean ±1 s.d. ( n =3). * P< 0.05, ** P< 0.01; Student’s t -test. Bar, 200 μm. ( c ) At the 4 d time point, neither IWP2 nor Snail1 excision interferes with stem cell exit from the pluripotent state as assessed by E-cadherin/Oct4 staining relative to untreated F/F controls. Bar, 200 μm. ( d ) Cardiomyocyte marker (cTnT) expression is upregulated at the RNA level following inhibition of Wnt signalling with IWP2 or Snail1 excision. cTnT mRNA expression levels are reported as the mean±1 s.d. ( n =3). * P <0.05, ** P <0.01; Student’s t -test. Bar, 200 μm. ( e ) cTnT protein levels are upregulated following IWP2 treatment or Snail1 excision. Immunofluorescent images are representative of three experiments performed. Full size image Recent studies have highlighted the divergent effects of Wnt signalling on mouse ESC function with effects ranging from promoting the maintenance of ESCs in a naive, pluripotent state to initiating EMT, differentiation and germ layer commitment [1] , [2] , [3] , [13] , [14] , [27] , [28] , [29] , [30] , [31] , [32] , [33] , [34] . Though Snail1 expression is likewise sensitive to Wnt regulation [10] , [12] , [13] , [15] , the roles played by Snail1 during ESC maintenance and differentiation have remained the subject of speculation. To date, virtually all predictions regarding the function of Snail1 in ESCs are based on a single study describing the generation of Snail1 KO mice [40] . In the absence of Snail1, embryonic development is curtailed at E7.5, yielding a completely penetrant, lethal phenotype [40] . The observed defects in gastrulation in vivo are, however, potentially consistent with altered ICM function, perturbations in cell cycle kinetics and cell survival or altered patterns of mesodermal cell migration arising as a consequence of a failure to downregulate E-cadherin efficiently. Our ability to detect Snail1 expression in the ICM of isolated blastocysts as well as in embryo-derived ESCs cultured in vitro lent support to the contention that Snail1 exerts upstream effects on stem cell function. In some respects, these results were unexpected as ESCs express high levels of E-cadherin, a prototypical gene target of Snail1-mediated transcriptional repression [15] , [16] . While the dual presence of Snail1 and E-cadherin distinguishes ESCs from inducible pluripotent stem cells that normally extinguish Snail1 expression during reprogramming [7] , [8] , Snail1 + /E-cadherin + populations have been identified previously in normal as well as neoplastic cells [57] , [58] . We considered the possibility that Snail1 might be functionally inactive as a consequence of post-translational phosphorylation, changes in nucleo-cytoplasmic trafficking or the ability to recruit DNA- or chromatin-modifying co-factors [15] , [16] . However, transcriptional profiling of Snail1-expressing versus -deleted ESCs support global effects on stem cell function, particularly with regard to metabolic cascades known to be activated in ESCs [59] . Interestingly, Snail1 has been reported to modulate glycolysis as well as oxidative phosphorylation in cancer cells [60] , [61] , raising the possibility that metabolic regulation reflects a conserved, EMT-independent function of the transcription factor in both normal and neoplastic cells. Nevertheless, despite the multiplicity of Snail1-regulated transcripts affected in naive stem cells, the key functions of self-renewal and pluripotency were left intact, thereby demonstrating that Wnt signalling does not require Snail1 to maintain the ESC ground state. Furthermore, our in vitro studies of ESC to EpiSC differentiation highlight the dispensability of Snail1 during the formation of EpiSCs. Nevertheless, efforts to assess the relative functions of wild-type versus Snail1 KO epiblasts in vivo will require further study. We would predict, however, that functional distinctions beyond pluripotency itself will likely result between the two populations given the numerous changes in gene transcription observed in Snail1 KO ESCs prior to EpiSC differentiation. In contrast with naive ESCs wherein Snail1 expression remains insensitive to Wnt signalling, EBs upregulate endogenous Wnt expression that triggers in turn a transient burst in Snail1 expression. Coincident with Snail1 expression, EBs decreased Nanog, Oct4 and Sox2 expression while downregulating E-cadherin and inducing mesenchymal cell markers. Each of these Wnt-dependent effects were blunted in Snail1-delected cells, but even in the absence of Snail1, EB differentiation proceeded to variably affected degrees by as yet undefined mechanisms that might be linked to the residual expression of Slug, Twist1 and Twist2, or the unabated expression of Zeb1 and Zeb2. Despite the ability of KO EBs to initiate differentiation, in the absence of Snail1 expression, a subpopulation of pluripotent cells could be identified with characteristics similar, if not identical, to EpiSCs, thereby supporting a required role for Snail1 in driving EpiSC exit and epiblast differentiation. Nevertheless, a subset of the KO cells were able to downregulate E-cadherin and differentiate into Flk1 + mesodermal cells. Further analyses demonstrated that while Snail1-independent programs can be initiated that support partial differentiation, the KO cells nevertheless display multiple defects in hematopoietic and cardiovascular development. Not surprisingly, GO analyses of KO ESCs and differentiating EBs display little overlap given the distinct roles of Snail1 in these divergent states. As such, though a requirement for Snail1 can be bypassed during stem cell-to-mesoderm commitment, the alternative programs that are mobilized to support lineage commitment do not allow for the progression of a fully realized differentiation programme. Interestingly, human ESCs also express Snail1 during their EMT-associated differentiation [1] . However, unlike mouse ESCs, human stem cells exhibit a more EpiSC-like status wherein Wnt signalling promotes, rather than inhibits, the germ layer commitment of distinct lineage-specified progenitors [62] . Despite these distinctions, we posit that Snail1 plays an equally important role in guiding Wnt-dependent, human ESC differentiation. Currently, the function of Wnt signalling in maintaining ESC/ICM function in vivo remains controversial [63] , [64] . By contrast, most accounts support the ability of Wnts to regulate adult stem cell pools in both normal and neoplastic states [17] , [65] . Cancer stem cells have been proposed to inappropriately co-opt ESC-like gene programs that confer tumour cells with self-renewal and pluripotent potential [9] , [15] , [16] , [21] , [22] , [23] , [25] , [26] . Further, forced overexpression of Snail1 or related EMT-associated transcription factors (including Slug, Twist1 and Zeb1) have been shown to promote cancer cells to adopt stem-like properties [9] , [15] , [16] , [21] , [22] , [23] , [25] , [26] . However, despite similarities between cancer stem cell and ESC signatures, we find that ESCs do not use Snail1 to maintain their naive status. Indeed, the expression of Snail1, Slug, Twist1 and Zeb1 all realize their highest level of expression when ESCs initiate differentiation and concomitantly lose their potential for self-renewal and pluripotency. Consistent with our findings in ESCs, recent studies indicate that cancer cells decrease—rather than increase—their stem-like qualities in tandem with the loss of their epithelial characteristics following the expression of Snail1 or related EMT-inducing transcription factors [58] , [66] , [67] , [68] . Though forced expression of Snail1 can support tumorsphere formation as well as changes in various cell surface markers (for example, CD44 and CD24) [9] , [22] , it remains uncertain as to whether these cell responses reflect, in and of themselves, the acquisition of true stem cell-like qualities. Our inability to link Snail1 expression in ESCs to self-renewal or pluripotency is also congruent with recent studies demonstrating that cancer stem cell signatures do not necessarily include the subset of gene products associate with cell stemness [69] . Likewise, transcription factors expressed in both ESCs and cancer stem cells (for example, TCF3) can function in diametrically opposed fashions in these two cell populations [70] . Apparently, despite a subset overlapping characteristics, ESCs and cancer stem cells appear to use Snail1 and other EMT-associated transcription factors in functionally distinct manners. Taken together, our studies describe new functions for Snail1 in regulating ESC functions that lie outside current paradigms. While Snail1 is expressed in ESCs, the transcription factor does not impact self-renewal, pluripotency, cell cycle kinetics, cell survival or EMT. Instead, Snail1 expression is linked to gene expression programs that encompass previously unappreciated roles for the transcription factor ( Fig. 7 ). Given the dynamic temporal pattern of endogenous Snail1 expression in normal ESCs—and possibly cancer cells—due caution should be exercised in interpreting results gleaned from studies using standard systems of overexpression. This issue notwithstanding, as ESCs subsequently initiate differentiation, Snail1 interfaces with Wnt-controlled programs that act downstream of early primitive streak formation to control neuroectodermal, mesodermal and endodermal lineage commitment decisions. During EB differentiation, Snail1-dependent EpiSC exit and E-cadherin repression clearly represent important arms of the developmental cascade. However, even in those EpiSC-derived populations that are able to bypass a requirement for Snail1-dependent EMT, the transcription factor plays a far broader role than appreciated previously in controlling the lineage fate determinations that define endothelial, hematopoietic and cardiomyocyte commitment ( Fig. 7 ). 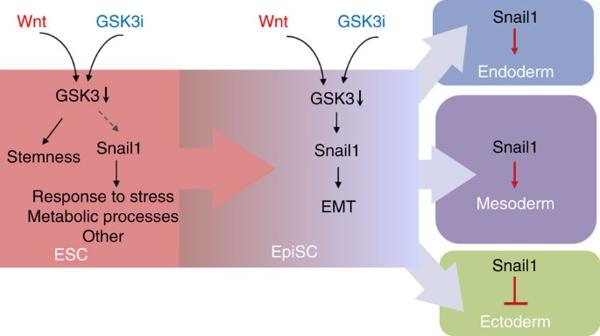Figure 7: Schematic of ESC Snail1 function. In ESCs, Wnt regulates stemness without affecting Snail1 expression whose functions are largely confined to metabolic control and stress responses. As ESCs exit their naive state, EpiSCs increase Snail1 expression via Wnt- and GSK3-dependent processes critical for driving the EMT programs that dictate endoderm, mesoderm and ectoderm commitment. Figure 7: Schematic of ESC Snail1 function. In ESCs, Wnt regulates stemness without affecting Snail1 expression whose functions are largely confined to metabolic control and stress responses. As ESCs exit their naive state, EpiSCs increase Snail1 expression via Wnt- and GSK3-dependent processes critical for driving the EMT programs that dictate endoderm, mesoderm and ectoderm commitment. Full size image Mice The Snai1 LacZ/+ ESCs were generated by the International Knockout Mouse Consortium (EUCOMM/KOMP) with the details described at the Consortium website (VG13025). Snai1 LacZ/+ mice were bred and maintained on a C57/B6 background. Mice carrying Snai1 fl/fl alleles [46] were bred with Tamoxifen-inducible CAG-Cre/Esr1* mice (Jackson Laboratory: 004453) to generate Snai1 fl/fl ; CAG-Cre+ conditional knockout mice. All protocols relating to this mouse work were reviewed and approved by the University of Michigan Committee on Use and Care of Animals. Isolation of blastocysts and derivation of ESCs E3.5 blastocysts were isolated from the uteri of pregnant C57/B6 female mice mated with Snai1 LacZ/+ male mice and fixed for X-gal staining. To derive Snai1 fl/fl ; CAG-Cre+ ESC lines, E3.5 blastocysts were collected from pregnant Snai1 fl/fl female mice that were mated with Snai1 fl/fl ; CAG-Cre+ male mice. ESCs were derived from blastocysts and cultured under standard conditions [10] . Axin2 LacZ/+ ESCs were provided by N. Russe (Stanford) [3] . ESC culture and embryoid body (EB) differentiation Snai1 fl/fl , CAG-Cre+ ESC lines were cultured atop feeder layers of mitomycin C-treated mouse embryonic fibroblasts in standard ESC culture medium (DMEM, 15% FBS; 1 × pen/strep; 4 mM glutamine, 50 μM β-mercaptoethanol; 1 × MEM non-essential amino acids, 1 × sodium pyruvate and 1,000 U ml −1 LIF). Medium changes were performed daily with ESCs passed every 2 days. For serum-free conditions, ESCs were cultured atop feeder layers in ESGRO-2i medium (SF016-100; Millipore). To generate Snail1 KO ESCs, Snai1 fl/fl ; CAG-Cre+ ESCs were treated with 100 nM 4-OHT for 2 d with untreated cells serving as the isogenic control. Each line of control and 4-OHT-treated ESCs were expanded and frozen for future use. To induce ESC differentiation, stem cells were recovered from feeder layers by trypsinization and seeded successively atop 0.1% gelatin-coated plastic dishes at 37 °C to remove contaminating fibroblasts. Embryoid bodies (EBs) were formed in differentiation media (ESC culture media with 10% FBS in the absence of LIF) in hanging droplets containing 2,000 feeder-free ESCs per 20 μl drop on petri dishes for 2 d. EBs were collected from the drops and cultured in ultralow attachment dishes in differentiation medium (counted as ‘day 0’), with the media being changed every 2 d. ESC to EpiSC differentiation ESCs were plated atop feeder layers in standard ESC culture medium for 24 h, the media replaced with EpiSC media (DMEM/F12, 20% knockout serum replacement, 4 mM glutamine, 100 μM β-mercaptoethanol, 1 × MEM non-essential amino acids, 12 ng ml −1 FGF2 and 20 ng ml −1 Activin A) for continuous culture. Medium changes were performed daily with cells passaged every 2-3 d as clumps using 0.5 mg ml −1 collagenase IV (17104-019; Invitrogen). The ROCK inhibitor, Y-27632 (1,254, Tocris), was added into the media during the first 24 h period after each passage [71] . After three passages, cells in EpiSC media were collected for RNA extraction or fixed and stained for alkaline phosphatase. Cell treatment ESCs or EBs were treated with either; LIF (ESG1106; 10 5 units per ml, Millipore), Wnt3a (GF160; 200 ng per ml, Millipore), CHIR99021 (04-0004, 3 μM, Stemgent), IWP2 (04-0034, 3 μM, Stemgent), FGF2 (100-18B; 10 ng per ml, Peprotech) or Activin A (120-14; 20 ng per ml, Peprotech). Immunofluorescence For ESC cultures, colonies cultured atop feeder layers were fixed in 4% PFA for 10 min at room temperature, washed with PBS and permeabilized with 0.2% Triton X-100/PBS for 5 min. After successive washes in PBS, the cells were blocked in 10 mg ml −1 BSA for 30 min and incubated with primary antibody for 1 h at room temperature. To assess relative immunofluorescent staining of E-cadherin, Nanog, Oct4 and Sox2, the intensity of individual colonies was determined with Molecular Dynamics ImageQuant 5.2 software and reported as the mean intensity per unit area. For EBs, spheroids were fixed in 4% PFA for 1 h on ice, followed by incubation in 30% sucrose/PBS at 4 °C overnight, and frozen in OCT (Tissue-Tek). Cryosections (10 μm) were washed in PBS for 5 min followed by permeabilization with 0.2% Triton X-100/PBS for 5 min. After washing in PBS, the samples were blocked in 10 mg ml −1 BSA for 30 min and incubated with primary antibody for 1 h at room temperature. Cells or slides were then washed three times with PBS for 5 min and incubated with secondary antibodies (Alexa 488 or 594-conjugated) for 1 h. The following primary antibodies were used for immunofluorescence; Nanog (rabbit; ab80892; 1:200, Abcam), Sox2 (rabbit; C70B1; 1:200, Cell Signaling), vimentin (mouse; 550513; 1:1,000, BD), Oct4 (rabbit; ab19857; 1:200, Abcam), E-Cadherin (mouse; 610181; 1:1,000, BD), N-Cadherin (mouse; 610920; 1:1,000, BD), fibronectin (rabbit; F3648; 1:1,000, Sigma), CD31 (rat; 553369; 1:1,000, BD), cardiac troponin T, (mouse; CT3; 1:1,000, DSHB) or βIII Tubulin (mouse; G7121; 1:1,000, Promega). Western blot and quantitative real-time PCR For western blotting, the following primary antibodies were used: Snail (mouse; L70G2, 1:1,000, Cell Signaling), E-Cadherin (mouse; 610181, 1:1,000, BD), β-actin (mouse, A1978, 1:5,000, Sigma). Densitometry of western blots was performed with Molecular Dynamics ImageQuant 5.2 software. Representative full-length images of western blots are shown in Supplementary Fig. 8 . Quantitative real-time PCR was performed using the power SYBR green PCR master mix (Applied Biosystems) according to the manufacturer’s instructions (primers are listed in Supplementary Table 1 ). LacZ staining and alkaline phosphatase (AP) staining For LacZ staining, ESCs, EBs or E3.5 blastocysts were fixed for 10 min at room temperature in buffer (0.2% gluteraldehyde, 0.1 M NaH 2 PO 4 , 5 mM EGTA, 2 mM MgCl 2 , 2% formaldehyde) followed by three, 5-min washes in rinse buffer (0.1 M NaH 2 PO 4 , 0.1% deoxycholic acid, 0.2% NP40 and 2 mM MgCl 2 ) and then incubated overnight in the dark at room temperature in staining buffer (1 mg ml −1 X-gal, 5 mM potassium ferricyanide and 5 mM potassium ferrocyanide in rinse buffer). For AP staining, ESC or EpiSC colonies were fixed for 2 min and incubated with an AP staining kit (Stemgent) following the manufacturer’s protocol. Relative AP staining intensity of 10 or more colonies in each experiment was determined with Molecular Dynamics ImageQuant 5.2 software. Flow cytometry EBs (4 d or 8-d-old) generated from F/F control or KO ESCs were dissociated with enzyme-free cell dissociation buffer (Invitrogen), resuspended in PBS and blocked by treatment with 1 μg of mouse IgG per 10 5 cells for 15 min at room temperature. The Fc-blocked cells were then incubated with FITC-conjugated anti-Flk1 (560680; BD) or PE-conjugated anti-E-cadherin (FAB7481P; R&D) (10 μl 1 −1 × 10 6 cells) for 45 min at 4 °C. Teratoma formation For ESCs injection, F/F control or KO ESCs were grown atop feeder layers and isolated by trypsinization and differential adhesion as described above. The single ESCs were resuspended in PBS (10 7 cells ml −1 ) with 10 6 cells injected subcutaneously into the hind limbs of 6-week-old male nude mice. For EB cell injection, 10-d-old F/F or KO EBs were either dissociated into single cells with non-enzymatic cell dissociation solution (Invitrogen) and injected into nude mice, or pools of whole EBs were mixed with Matrigel and injected into NOD scid gamma mice [48] . Teratoma growth was assessed weekly and the tumours collected after 6 weeks either for RNA isolation or paraffin embedding, sectioning and histological staining. Expression array profiling and analysis Total mRNA was collected and purified using RNeasy Mini Kits (QIAGEN) [46] . Sample quality was confirmed using a Bioanalyzer 2100 and all samples profiled on Affymetrix Mouse MG-430 PM expression array strips. Expression values for each probe set were calculated using the robust multi-array average (RMA) system [46] and filtered for genes with a fold change greater than twofold. Heatmaps of selected gene lists were generated using Gene Cluster 3.0 and TreeView 1.6 (ref. 46 ) Gene ontology analysis was performed using MetaCore from Thomson Reuters (version 6.11, build 41105). For miRNA array, total mRNA was collected from EBs using a mirVana miRNA isolation kit (Life Technologies) and performed using TaqMan MicroRNA panels OpenArray (Life Technologies). Statistical analysis All data are presented as the mean±s.d. of three or more independent experiments. Significance was determined by Student’s t -test or ANOVA assay. Accession codes: Microarray data has been deposited in GEO under accession numbers GSE53106 , GSE53107 , and GSE53108 . How to cite this article: Yongshun, L. et al. Snail1-dependent control of embryonic stem cell pluripotency and lineage commitment. Nat. Commun. 5:3070 doi: 10.1038/ncomms4070 (2014).